ATM kinase sustains HER2 tumorigenicity in breast cancer ATM kinase preserves genomic stability by acting as a tumour suppressor. However, its identification as a component of several signalling networks suggests a dualism for ATM in cancer. Here we report that ATM expression and activity promotes HER2-dependent tumorigenicity in vitro and in vivo . We reveal a correlation between ATM activation and the reduced time to recurrence in patients diagnosed with invasive HER2-positive breast cancer. Furthermore, we identify ATM as a novel modulator of HER2 protein stability that acts by promoting a complex of HER2 with the chaperone HSP90, therefore preventing HER2 ubiquitination and degradation. As a consequence, ATM sustains AKT activation downstream of HER2 and may modulate the response to therapeutic approaches, suggesting that the status of ATM activity may be informative for the treatment and prognosis of HER2-positive tumours. Our findings provide evidence for ATM’s tumorigenic potential revising the canonical role of ATM as a pure tumour suppressor. ATM kinase is a major guardian of genomic stability due to its central role in DNA damage response (DDR) elicited by double-stranded breaks [1] . ATM was originally identified as the product of the gene mutated in Ataxia Telangiectasia (A-T), a rare recessive genetic disorder characterized by several features including cerebellar neurodegeneration and immunological disorders [2] . A-T patients are also characterized by an increased predisposition to develop malignancies, in particular lymphoma and leukaemia, consistent with the central role of ATM in DDR (reviewed in ref. 3 ). Accordingly, ATM expression is aberrantly low in many lymphomas [4] , [5] . Moreover, ATM heterozigosity has been linked to an increased risk in the occurrence of solid tumours, in particular breast cancer [6] , [7] , [8] , some ATM mutations may confer breast cancer susceptibility [9] , [10] while comprehensive sequencing of ATM identified a preferential ATM loss of function in familial breast cancer patients compared with healthy controls [11] . Such in vivo evidence strongly supports the notion that ATM is a tumour suppressor gene consistent with its central role in the prevention of genomic instability. However, the identification of ATM as part of several signalling pathways significantly activated in neoplastic cells, raised the question whether ATM function in cancer may be more complex than expected. Indeed, ATM activity may promote cell growth and proliferation [12] , protein synthesis [13] , insulin receptor and MET receptor prosurvival and proliferative signals [14] , [15] and AKT activity [16] , [17] . Furthermore, ATM has been identified as a modulator of hypoxia response as it promotes HIF-1α protein stabilization [18] and enhances tumour angiogenesis [19] as well, being a novel modulator of glucose metabolism and of mitochondrial functionality [20] , both of which are aberrantly modified in cancer. HER2 positivity is identified in 15–20% of primary human breast cancers and is associated with an aggressive tumour type with poor survival [21] . The introduction of Trastuzumab (Herceptin), the humanized monoclonal antibody (mAb) against HER2 has completely changed the history of HER2+ breast cancer patients both in terms of time to recurrence and survival [22] , although the development of resistance to this treatment is still a major problem. HER2 belongs to the family of HER receptors and its aberrant activation in cancer is mainly due to gene amplification and overexpression (reviewed in refs 23 , 24 ). As a consequence, HER2 promotes cell transformation [25] , [26] and elicits the constitutive activation of a panel of downstream signalling molecules including PI3K, SRC, AKT and MAPKs (reviewed in refs 23 , 24 ). Interestingly, it has been recently shown that ATM is phosphorylated on Ser1981 in a somatic mouse model of breast cancer dependent on the expression of HER2 (ERBB2/NeuN) receptor tyrosine kinase [27] . Although the functional significance of ATM phosphorylation (ATM-p) on Ser1981 in this context has not been fully elucidated [27] , the authors, given the identification of ATM phosphorylation on Ser1981 as a marker of ATM kinase activation in response to several stimuli [28] , propose that, in this context ATM is activated as part of the DDR to counteract tumour progression [27] as previously reported (reviewed in ref. 29 ). However, the identification of ATM activation downstream of other receptor tyrosine kinases (RTKs) [14] , [15] , together with its role in sustaining tumorigenic signals such as AKT activation [16] , [17] , suggest that, alternatively, HER2-positive tumours may represent an intriguing model system for testing the significance of ATM activity in this context and assay the hypothesis that it may differently modulate tumour progression depending on the specific signalling networks that sustain tumorigenicity. Here we show that ATM expression and activity sustains HER2 expression, enhancing its protein stability and promoting its downstream signalling. Surprisingly, ATM inhibition selectively impairs HER2-dependent tumorigenicity in vitro and in vivo , suggesting that in this context its activity may promote tumour progression. Importantly, ATM phosphorylation in HER2+ tumours identifies a subclass of patients characterized by significantly reduced disease-free survival (DFS). ATM promotes transformation of HER2-positive cancer cells The observation that ATM kinase may be induced downstream of RTKs and may sustain AKT activation raised the question as to whether in particular contexts ATM may promote tumorigenesis. To test our hypothesis, we developed in vitro and in vivo models based on breast cancer cell lines overexpressing HER2. We first evaluated ATM’s contribution to HER2-dependent neoplastic transformation by evaluating the anchorage-independent growth of SKBR3 cells, a well-characterized in vitro model derived from a HER2-positive breast cancer patient, in the presence or absence of ATM activity and expression. Surprisingly, soft-agar assays showed that colony formation was significantly suppressed upon incubation with a specific inhibitor of ATM kinase activity, KU-55933, as well as by stable interference for ATM expression (shATM#1 and shATM#3) relative to their respective controls, similar to what we observed upon HER2 expression interference ( Fig. 1a,b ). Accordingly, we could show that ATM phosphorylation on Ser1981-ATM (ATM-p) in SKBR3 cells is abrogated by treatment with specific inhibitor of ATM kinase activity, KU-55933, as well as by treatment with Trastuzumab (Herceptin), a mAb successfully used in clinics for HER2-positive breast cancer treatment selectively targeting HER2 (ref. 22 ) ( Supplementary Fig. 1 ). Similar results were also obtained in other HER2-positive cancer cell lines ( Supplementary Fig. 2A,B ). Conversely, in cell lines that do not overexpress HER2 (MCF7, T47D and MDA-MB-231), the ability to grow in soft agar was unaffected by specific short hairpin RNA (shRNA) against ATM messenger RNA ( Fig. 1c ; Supplementary Fig. 2C,D ). Interestingly, the stable ectopic overexpression of HER2 in the MCF7 context was sufficient to promote MCF7-HER2 cell growth in soft agar’s dependence on ATM ( Fig. 1c ). 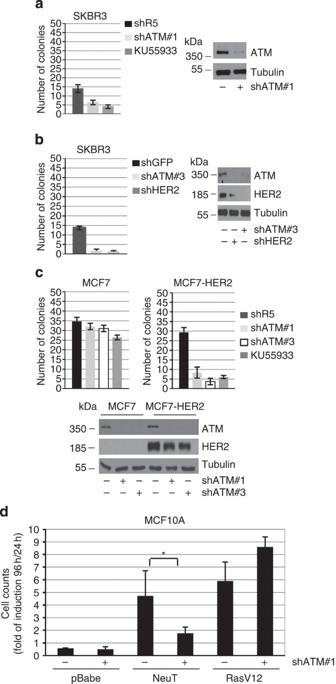Figure 1: ATM expression and activity promotes HER2 tumorigenicityin vitro. (a–c) Anchorage-independent growth of HER2+ (SKBR3), HER2− (MCF7), exogenous HER2+ (MCF7-HER2) breast cancer cell lines treated with ATM kinase inhibitor KU-55933 10 μM (a,c), infected with retrovirus or expressing specific RNA interference for ATM (shATM#1) or a control sequence (shR5, labelled as −), or infected with lentivirus expressing RNA interference for ATM (shATM#3), for HER2 (shHER2) or a control sequence (shGFP, labelled −) (b). Colonies are counted after 10 days and represented as mean±s.d. (n=6 for each condition). The panels on the bottom display representative western blots. (d) ATM interference selectively impairs NeuT-driven transformation in human mammary gland epithelial cells, MCF10A. Cell proliferation assay in MCF10A-pBabe, MCF10A-NeuT and MCF10A-RasV12 cell lines infected with a lentiviral construct expressing ATM shRNA interference sequence or control shRNA interference sequence. Bars display the cell number for each cell line counted 96 h after seeding; this number has been normalized on cell number counted 24 h after seeding. Cell numbers have been counted in triplicate in three independent experiments for each condition. Data are shown as mean+s.d. (*Pvalue for NeuT versus NeuT-shATM=0.03;Pvalues were calculated using two-sided Studentt-tests). Figure 1: ATM expression and activity promotes HER2 tumorigenicity in vitro . ( a – c ) Anchorage-independent growth of HER2+ (SKBR3), HER2− (MCF7), exogenous HER2+ (MCF7-HER2) breast cancer cell lines treated with ATM kinase inhibitor KU-55933 10 μM ( a , c ), infected with retrovirus or expressing specific RNA interference for ATM (shATM#1) or a control sequence (shR5, labelled as −), or infected with lentivirus expressing RNA interference for ATM (shATM#3), for HER2 (shHER2) or a control sequence (shGFP, labelled −) ( b ). Colonies are counted after 10 days and represented as mean±s.d. ( n =6 for each condition). The panels on the bottom display representative western blots. ( d ) ATM interference selectively impairs NeuT-driven transformation in human mammary gland epithelial cells, MCF10A. Cell proliferation assay in MCF10A-pBabe, MCF10A-NeuT and MCF10A-RasV12 cell lines infected with a lentiviral construct expressing ATM shRNA interference sequence or control shRNA interference sequence. Bars display the cell number for each cell line counted 96 h after seeding; this number has been normalized on cell number counted 24 h after seeding. Cell numbers have been counted in triplicate in three independent experiments for each condition. Data are shown as mean+s.d. ( *P value for NeuT versus NeuT-shATM=0.03; P values were calculated using two-sided Student t -tests). Full size image It has been previously shown that ATM deficiency may result in a strong impairment of cell proliferation [12] . In agreement with this observation, we demonstrate here that the genetic interference of ATM significantly delays cellular growth in all cell lines assayed in our study ( Supplementary Fig. 3 ). As ATM downregulation selectively enhances transformation of only the cell lines we assayed characterized by HER2 overexpression, we suggest that the ability of ATM to modulate cell proliferation is not sufficient to predict its effect on cell transformation. To further clarify whether ATM expression selectively promotes HER2-dependent tumorigenicity, we transformed MCF10A cells, an established normal human mammary gland epithelial cellular system, with constitutively active forms of HER2 (NeuV664E, named NeuT) or Ras (RasG12V, named RasV12) as previously described [30] . As expected, NeuT as well RasV12 expression trigger cell transformation, so allowing these cells to grow in the absence of serum and mitogens (1% FBS) as compared with control cells, which are not transformed and therefore unable to grow in such conditions ( Fig. 1d ). Significantly, when ATM expression was genetically inhibited by specific shRNA interference ( Supplementary Fig. 4A ), MCF10A-NeuT-shATM cells lost the transformed phenotype ( Fig. 1d ). The inhibition of ATM expression ( Supplementary Fig. 4B ) did not dampen MCF10-RasV12 cells’ ability to grow in 1% FBS, suggesting that ATM expression is specifically required for HER2-driven transformation at least in this cellular system ( Fig. 1d ). ATM sustains HER2-dependent tumorigenicity in vivo To evaluate the requirement of ATM in HER2-triggered tumour growth in vivo , we compared the tumorigenic potential of MCF7-HER2 cells stably interfered for ATM expression (or not) in nude mice xenograft experiments. Remarkably, we found that tumour growth, caused by subcutaneous injection of MCF7-HER2-shATM cells, was significantly diminished compared with that induced by MCF7-HER2 control cells ( Fig. 2a–c ). shATM led to a statistically significative four- to fivefold reduction in tumour size reduction in tumour at 4 weeks after injection ( Fig. 2a–c ). Conversely, ATM interference in MCF7 cells promoted their ability to drive tumour growth in nude mice ( Supplementary Fig. 5 ), supporting the idea that ATM may selectively sustain HER2 tumorigenicity in vivo . 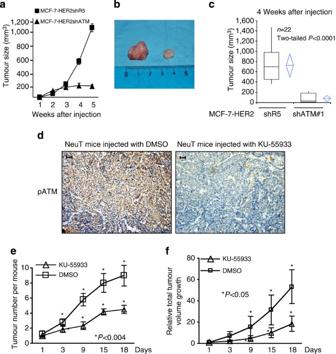Figure 2: ATM expression and activity promotes HER2 tumorigenicityin vivo. (a–c) MCF7-HER2shR5 and MCF7-HER2shATM cells were subcutaneously injected into nude mice and tumour growth was monitored. (a) Quantification of tumour size during 5 weeks of xenograft growth. (b) Pictures representative of tumours after dissection. (c) Comparison of tumour size between MCF7-HER2shR5 and MCF7-HER2shATM xenografts. Each plot graphically shows the central location and scatter/dispersion of the values of each group: the line series in the rectangular shaped box indicate the median value of the data and the end of vertical lines indicates the minimum and the maximum data value. The mean and its confidence interval are shown in the diamond shape box.Pvalue was calculated according to independent samplest-test (n=22). (d–f) FBV-NeuT mice were intraperitoneally injected with 10 mg kg−1KU-55933 in DMSO or with DMSO as control, every 2 days for 2 weeks starting from the appearance of the first mammary tumour, and sacrificed 3 days after the last injection. ATM-p was revealed by immunohistochemistry on tumours, scale bars, 30 μm (d). Tumour growth curves showing delayed tumour onset and reduced tumour incidence (e) and reduced relative tumour volume growth (f) of KU-55933-injected mice versus DMSO control mice. Data are shown as mean+s.d. (* indicates thePvalue for KU-55933 versus DMSO;Pvalues were calculated using two-sided Student’st-tests). Figure 2: ATM expression and activity promotes HER2 tumorigenicity in vivo . ( a – c ) MCF7-HER2shR5 and MCF7-HER2shATM cells were subcutaneously injected into nude mice and tumour growth was monitored. ( a ) Quantification of tumour size during 5 weeks of xenograft growth. ( b ) Pictures representative of tumours after dissection. ( c ) Comparison of tumour size between MCF7-HER2shR5 and MCF7-HER2shATM xenografts. Each plot graphically shows the central location and scatter/dispersion of the values of each group: the line series in the rectangular shaped box indicate the median value of the data and the end of vertical lines indicates the minimum and the maximum data value. The mean and its confidence interval are shown in the diamond shape box. P value was calculated according to independent samples t -test ( n =22). ( d – f ) FBV-NeuT mice were intraperitoneally injected with 10 mg kg −1 KU-55933 in DMSO or with DMSO as control, every 2 days for 2 weeks starting from the appearance of the first mammary tumour, and sacrificed 3 days after the last injection. ATM-p was revealed by immunohistochemistry on tumours, scale bars, 30 μm ( d ). Tumour growth curves showing delayed tumour onset and reduced tumour incidence ( e ) and reduced relative tumour volume growth ( f ) of KU-55933-injected mice versus DMSO control mice. Data are shown as mean+s.d. (* indicates the P value for KU-55933 versus DMSO; P values were calculated using two-sided Student’s t -tests). Full size image To further ascertain whether ATM counteracts HER2 tumorigenicity in vivo , we adopted a transgenic mouse model expressing rat HER2/neu oncogene in the mammary gland. In these mice, mammary tumours develop spontaneously 15 weeks after birth [31] . Immunohistochemistry revealed that ATM is phosphorylated on S1981 in these mammary tumours ( Fig. 2d ; Supplementary Table 1 ) consistently with ATM activation in breast cancer cell lines derived from human patients overexpressing HER2 ( Supplementary Fig. 1 ). We show that in vivo administration of KU-55933 by intraperitoneal injection in wild-type mice does not exert major toxicity and is sufficient to downregulate ATM phosphorylation induced by ionizing radiation ( Supplementary Fig. 6 ); the implication is that KU-55933 can be used in vivo to downregulate endogenous ATM activation. NeuT mice were injected intraperitoneally with KU-55933 every 2 days for 2 weeks, starting immediately after the development of the first tumour; tumour growth was monitored at the indicated times. Mice injected with KU-55933 showed reduced multiplicity and decreased total tumour volume compared with control animals injected with dimethylsulphoxide ( Fig. 2e,f ). Interestingly, immunohistochemistry analysis revealed that tumours developed in KU-55933-treated animals were significantly impaired for ATM-p on Ser1981 ( Fig. 2d ; Supplementary Table 1 ). This confirms that KU-55933 treatment downregulates endogenous ATM activity, thus impinging on HER2 tumorigenicity. Overall, these findings indicate that, functional ATM kinase is required to support HER2-dependent tumorigenesis. ATM phosphorylation and expression sustains HER2 protein levels We then sought to elucidate the molecular mechanism through which ATM modulates HER2 tumorigenicity. Surprisingly, we observed that inhibition of ATM kinase activity upon treatment with KU-55933 significantly decreased NeuT expression in vivo ( Fig. 3a ; Supplementary Table 2 ). Consistently, KU-55933 significantly decreased HER2 protein levels in SKBR3 as well as in SKOV3 cells, as revealed by immunoblotting analysis ( Fig. 3b,c ). Similar results were obtained in cells where we genetically downregulated ATM expression by specific RNA interference (shATM#1, Fig. 3d ). Accordingly, interference of ATM expression caused a marked reduction in HER2 protein levels expressed on the cell surface ( Fig. 3e ), supporting the conclusion that ATM expression sustains endogenous HER2 protein levels. Interestingly, the downregulation of ATM expression also triggered a decrease in HER2 protein levels in MCF7-HER2 cells, derived from MCF7 cells stably transfected with HER2. This suggests that ATM also impinges on exogenously expressed HER2 expression, therefore, independently of its transcription ( Fig. 3f ). 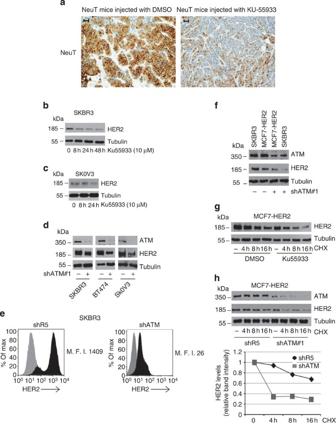Figure 3: ATM kinase regulates HER2 receptor levels and stability. (a) NeuT levels were revealed by immunohistochemistry on tumours from NeuT mice injected with 10 mg kg−1KU-55933 in DMSO or with DMSO as inFig. 2d, scale bars, 30 μm. (b,c) Western blot experiments showing HER2 receptor protein levels in SKBR3 cell line and SKOV3 cell line upon treatment with ATM inhibitor KU-55933 (10 μM for the indicated times). (d) Western blot for detection of HER2 receptor levels in HER2+ breast cancer cell line stably infected with retrovirus expressing control (shR5, labelled −) or ATM RNA interference (shATM#1, labelled +). (e) Representative histograms showing flow cytometry analysis of HER2 expression on cell surface. Incubation with phycoerythrin-conjugated goat anti-mouse IgG alone served as negative controls (isotype, grey solid histograms). MFI, mean fluorescence intensity. (f) Western blot for detection of HER2 and ATM in the indicated cell lines stably infected with retrovirus expressing control (shR5, labelled −) or ATM RNA interference (shATM#1, labelled +). (g) Representative western blot showing HER2 protein degradation upon treatment with KU-55933 (10 μM) for 16 h and subsequently inhibition of protein synthesis with cycloheximide (100 μg ml−1) for indicated times. (h) Representative western blot (upper panel) and quantification (lower panel) of HER2 protein degradation in MCF7-HER2shR5 cell line compared with MCF7-HER2shATM. CHX, cycloheximide (100 μg ml−1). Figure 3: ATM kinase regulates HER2 receptor levels and stability. ( a ) NeuT levels were revealed by immunohistochemistry on tumours from NeuT mice injected with 10 mg kg −1 KU-55933 in DMSO or with DMSO as in Fig. 2d , scale bars, 30 μm. ( b , c ) Western blot experiments showing HER2 receptor protein levels in SKBR3 cell line and SKOV3 cell line upon treatment with ATM inhibitor KU-55933 (10 μM for the indicated times). ( d ) Western blot for detection of HER2 receptor levels in HER2+ breast cancer cell line stably infected with retrovirus expressing control (shR5, labelled −) or ATM RNA interference (shATM#1, labelled +). ( e ) Representative histograms showing flow cytometry analysis of HER2 expression on cell surface. Incubation with phycoerythrin-conjugated goat anti-mouse IgG alone served as negative controls (isotype, grey solid histograms). MFI, mean fluorescence intensity. ( f ) Western blot for detection of HER2 and ATM in the indicated cell lines stably infected with retrovirus expressing control (shR5, labelled −) or ATM RNA interference (shATM#1, labelled +). ( g ) Representative western blot showing HER2 protein degradation upon treatment with KU-55933 (10 μM) for 16 h and subsequently inhibition of protein synthesis with cycloheximide (100 μg ml −1 ) for indicated times. ( h ) Representative western blot (upper panel) and quantification (lower panel) of HER2 protein degradation in MCF7-HER2shR5 cell line compared with MCF7-HER2shATM. CHX, cycloheximide (100 μg ml −1 ). Full size image To ascertain whether ATM modulates HER2 protein stability, we tested whether the downregulation of ATM kinase activity or expression accelerates HER2 protein degradation by blocking nascent translation with cycloheximide (CHX). ATM pharmacological inhibition triggered the downregulation of HER2 protein basal levels ( Fig. 3g ) and slightly enhanced HER2 degradation upon CHX treatment ( Fig. 3g ). In line with this finding, ATM interference reduced the basal levels of HER2 protein ( Fig. 3h ) and accelerated HER2 protein degradation, as HER2 protein levels were markedly reduced already after 4 h treatment with CHX, compared with control cells ( Fig. 3h ). Overall, we can conclude that HER2 protein stability is significantly enhanced by ATM kinase expression and activity. ATM inhibition triggers HER2 ubiquitination and degradation The protein stability of HER2 is strictly modulated by its interaction with the HSP90 chaperone machinery. This interaction is fundamental for preventing HER2 ubiquitination and degradation. Disruption of this protein–protein interaction has been proposed as a valuable therapeutic strategy to target HER2-dependent tumorigenesis (reviewed in ref. 32 ). To test whether ATM expression and activity modulates HER2–HSP90 interaction, HER2 was immunoprecipitated from MCF7-HER2 cells; coimmunoprecipitated HSP90 was revealed by specific antibodies. Importantly, HER2–HSP90 interaction was markedly decreased by ATM expression downregulation upon specific shRNA interference as well as by the inhibition of ATM kinase activity, at the same extent obtained upon incubation with 17AAG, a well-known inhibitor of HSP90, which disrupts the ability of HSP90 to interact with its client proteins ( Fig. 4a ). The same results were also obtained in SKBR3 cells endogenously overexpressing HER2 ( Fig. 4b ; Supplementary Fig. 7A ). ATM downregulation resulted in a strong induction of both exogenous and endogenous HER2 protein ubiquitination both in MCF7-HER2 and in SKBR3 cells ( Fig. 4c,d ). This supports the hypothesis that ATM promotes HER2–HSP90 complex and therefore prevents HER2 ubiquitination and degradation. Accordingly, transient transfection of HER2 in HEK293 cells may trigger ATM activation and its recruitment to a ternary complex HER2–HSP90–ATM ( Supplementary Fig. 7B,C ). 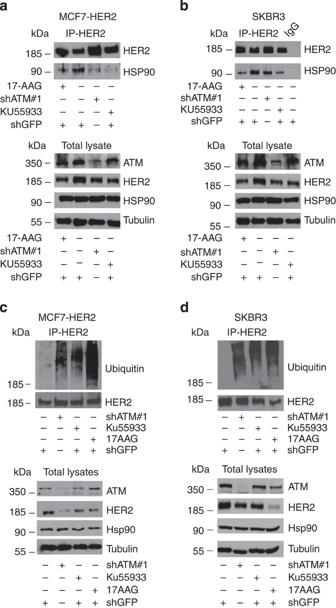Figure 4: ATM inhibition induces dissociation of HER2 from HSP90, followed by ubiquitination and degradation of HER2 in breast cancer cells. (a–d) Cellular extracts from MCF7-HER2 (a,c) and SKBR3 cell lines (b,d) were prepared for immunoprecipitation with anti-HER2 antibody and subjected to western blotting with anti-HSP90 (a,b) and anti-ubiquitin antibodies (c,d). Cells were infected with retrovirus expressing shATM RNA interference or shGFP as control or treated with ATM kinase inhibitor KU-55933 (10 μM for 24 h). HSP90 inhibitor, 17AAG (1 μM for 2 h), was used as a positive control. Western blots on total extracts were carried out loading the same amount of total proteins for each sample to assess the effect of the different treatments on HER2 protein levels. Tubulin has been used as a loading control. Dissociation of HSP90 from HER2 and HER2 ubiquitination were revealed after immunoprecipitation carried out upon normalization of the HER2 protein levels to ensure that the reduction in the amount of HSP90-interacting protein upon treatments was independent of the decrease in HER2 protein levels. Figure 4: ATM inhibition induces dissociation of HER2 from HSP90, followed by ubiquitination and degradation of HER2 in breast cancer cells. ( a – d ) Cellular extracts from MCF7-HER2 ( a , c ) and SKBR3 cell lines ( b , d ) were prepared for immunoprecipitation with anti-HER2 antibody and subjected to western blotting with anti-HSP90 ( a , b ) and anti-ubiquitin antibodies ( c , d ). Cells were infected with retrovirus expressing shATM RNA interference or shGFP as control or treated with ATM kinase inhibitor KU-55933 (10 μM for 24 h). HSP90 inhibitor, 17AAG (1 μM for 2 h), was used as a positive control. Western blots on total extracts were carried out loading the same amount of total proteins for each sample to assess the effect of the different treatments on HER2 protein levels. Tubulin has been used as a loading control. Dissociation of HSP90 from HER2 and HER2 ubiquitination were revealed after immunoprecipitation carried out upon normalization of the HER2 protein levels to ensure that the reduction in the amount of HSP90-interacting protein upon treatments was independent of the decrease in HER2 protein levels. Full size image ATM modulates HER2 + cell sensitivity to therapeutic agents The therapeutical use of Trastuzumab (Herceptin), a mAb counteracting HER2 tumorigenicity, significantly improved HER2-positive breast cancer treatment. However, a major problem is that the lack of comprehension of the molecular mechanisms promoting resistance or acquired resistance, significantly reduces this treatment’s success rate. Sensitivity is strictly dependent on HER2 high expression and has been mainly linked to an inhibitory effect of Trastuzumab on cell proliferation [33] , [34] , [35] . Accordingly we show that HER2-overexpressing cells where ATM has been downregulated by specific shRNA interference became significantly resistant to Trastuzumab; this further supports the conclusion that ATM sustains HER2 expression, required for efficient targeting ( Fig. 5a ). Interestingly, it has been suggested that HER2 aberrant expression may negatively affect ER+ cell sensitivity to tamoxifen [36] , [37] . Using the same experimental system, we were able to confirm that estrogen receptor positive (ER+) MCF7 cells that express very low levels of endogenous HER2 are highly sensitive to tamoxifen, independently of ATM expression ( Fig. 5b ). Conversely, according to previous reports [36] , [37] , the overexpression of HER2 triggers tamoxifen resistance in MCF7-HER2 cells ( Fig. 5b ). It is noteworthy that ATM inhibition restores MCF7-HER2 cells sensitivity to tamoxifen, providing functional evidence for shATM-dependent downregulation of HER2 expression ( Fig. 5b ). 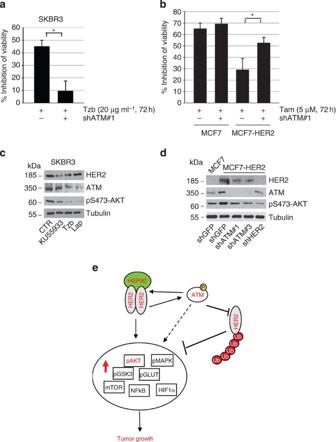Figure 5: ATM modulates HER2-positive cell sensitivity to therapeutic approaches. (a) Viability assay represented in the histogram as mean±s.d. (n=6). SKBR3shR5 control cell lines and SKBR3shATM were incubated or not in the presence of Trastuzumab (Tzb, 20 μg ml−1for 72 h). Viability was assessed with the Cell Titer Glo Luminescent Assay and represented as the percentage of inhibition of viability measured in cells treated without Tzb.*Pvalue for SKBR3shR5 versus SKBR3shR5+Tzb=0.001;Pvalues were calculated using two-sided Student’st-tests. (b) Viability assay represented in the histogram as mean±s.d. (n=3 for each condition). MCF7 and MCF-7HER2, interfered or not for ATM expression, were incubated (or not) in the presence of Tamoxifen (Tam 5 μM for 72 h). Viability was assessed as inaand represented as the percentage of inhibition of viability measured in cells treated without Tam (*Pvalue=0.002). (c,d) Representative western blot showing phosphorylation of AKT on S473 (pS473-AKT) upon treatment with KU-55933 (10 μM for 48 h) or Trastuzumab (Tzb, 20 μg ml−1for 48 h) or Lapatinib (100 mM, for 48 h) (a) and upon infection with lentiviruses expressing shATM#1 or shATM#3 or shHER2 RNA interference or shGFP as control (b). (e) Proposed model depicting the interplay between HER2 and ATM kinase. ATM stabilizes HER2 protein enhancing HER2 interaction with HSP90, thus preventing HER2 ubiquitination and degradation. HER2 may promote the activation of several tumorigenic pathways (red arrow). ATM supports HER2’s ability to activate AKT signaling. Future experiments will clarify whether ATM directly modulates other HER2 signaling (black labels) dependently on or independently of its effect on HER2 (dashed arrow). Figure 5: ATM modulates HER2-positive cell sensitivity to therapeutic approaches. ( a ) Viability assay represented in the histogram as mean±s.d. ( n =6). SKBR3shR5 control cell lines and SKBR3shATM were incubated or not in the presence of Trastuzumab (Tzb, 20 μg ml −1 for 72 h). Viability was assessed with the Cell Titer Glo Luminescent Assay and represented as the percentage of inhibition of viability measured in cells treated without Tzb. *P value for SKBR3shR5 versus SKBR3shR5+Tzb=0.001; P values were calculated using two-sided Student’s t -tests. ( b ) Viability assay represented in the histogram as mean±s.d. ( n =3 for each condition). MCF7 and MCF-7HER2, interfered or not for ATM expression, were incubated (or not) in the presence of Tamoxifen (Tam 5 μM for 72 h). Viability was assessed as in a and represented as the percentage of inhibition of viability measured in cells treated without Tam ( *P value=0.002). ( c , d ) Representative western blot showing phosphorylation of AKT on S473 (pS473-AKT) upon treatment with KU-55933 (10 μM for 48 h) or Trastuzumab (Tzb, 20 μg ml −1 for 48 h) or Lapatinib (100 mM, for 48 h) ( a ) and upon infection with lentiviruses expressing shATM#1 or shATM#3 or shHER2 RNA interference or shGFP as control ( b ). ( e ) Proposed model depicting the interplay between HER2 and ATM kinase. ATM stabilizes HER2 protein enhancing HER2 interaction with HSP90, thus preventing HER2 ubiquitination and degradation. HER2 may promote the activation of several tumorigenic pathways (red arrow). ATM supports HER2’s ability to activate AKT signaling. Future experiments will clarify whether ATM directly modulates other HER2 signaling (black labels) dependently on or independently of its effect on HER2 (dashed arrow). Full size image HER2 overexpression triggers the aberrant activation of several signalling pathways that, taken together, lead to tumorigenesis [23] , [24] . The induction of AKT phosphorylation has been clearly linked to sustained cell proliferation and tumorigenicity; specific compounds, including Trastuzumab and Lapatinib, which target the kinase activity of HER2 and EGF receptor, may interfere with this signalling [33] , [34] , [35] . We therefore set out to investigate whether ATM inhibition might also result in the modulation of AKT phosphorylation. We discovered that the interference of ATM expression together with the inhibition of ATM kinase activity, caused the downregulation of HER2 protein levels and the inhibition of AKT activation in SKBR3 cells, similarly to what was observed upon Trastuzumab or Lapatinib treatment ( Fig. 5c ). A similar result was also obtained in MCF7-HER2 cells, using two shRNA interferences specific for ATM expression ( Fig. 5d ). Intriguingly, we found that HER2 may promote ATM protein expression levels ( Fig. 5c,d ), suggesting the occurrence of a positive feedback loop. Overall, these data indicate that ATM regulates HER2 expression and functionality ( Fig. 5e ). ATM-p predicts worse DFS in HER2 + human breast cancer To further uncover the complexity of ATM’s role in breast cancer progression, we sought to evaluate the occurrence of ATM activation as revealed by immunostaining with specific anti-pS1981-ATM antibodies (ATM-p) in a retrospective series of 167 patients diagnosed with invasive breast cancer ( Supplementary Fig. 7 ; Supplementary Table 2 ). Eighty-seven patients were HER2 positive and 80 HER2 negative. None of the HER2-positive patients included in this study were submitted to trastuzumab or other any anti-HER2 treatment. In our series, 59% of the tumours stained positive for ATM phosphorylation on S1981, ATM-p ( Supplementary Table 3 ). No significant correlation ( χ 2 -test) was observed between ATM-p positivity and tumour size ( P =0.354) and lymph node status ( P =0.091). Conversely, immunohistochemistry (IHC) expression of ATM-p was directly related to the tumour-grading ( P =0.001) proliferation index assessed by Ki67 staining ( P =0.001), HER2 positivity ( P =0.019) and hormonal receptor negativity ( P =0.005 and P =0.023) ( Table 1 ). We then set out to investigate whether IHC expression of ATM-p is differently associated with disease progression in HER2+ or HER2− breast cancer patients. Analysing our series of 167 cases by unadjusted Kaplan–Meier curves, we observed that the association of ATM-p and HER2 positivity significantly affects disease free survival (DFS), ( P =0.001, long-rank test). As illustrated in Fig. 6 , ATM-p positive/HER2-positive breast cancer (BC) patients have the shortest DFS (42.5%) than those with ATM-p-negative/HER2-positive (78.1%) and ATM-p-negative/HER2-negative BC (96.9%). Univariate analysis (Cox model) further confirmed these data, identifying lymph node positivity ( P =0.013), ER/PgR ( P =0.001 and 0.041) negativity, HER2 overexpression ( P =0.001), high proliferation index Ki67 ( P =0.002) and ATM-p positivity ( P =0.001) as significant predictors of worse DFS ( Supplementary Table 4 ). Overall, these data suggest that the identification of ATM phosphorylation on Ser1981 by IHC may have a prognostic and therapeutic significance. Table 1 Relationship between ATM-p expression and clinicopathological parameters. 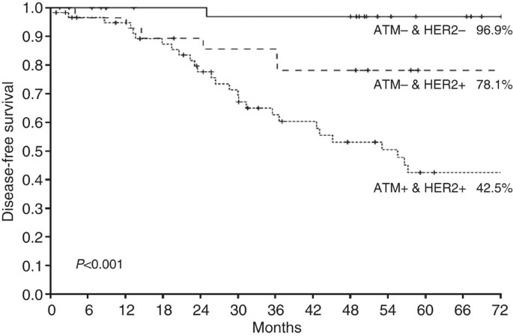Figure 6: Kaplan–Meier estimates of disease-free survival for ATM-p/HER2 status. Kaplan–Meier curves in a series of 167 HER2-negative and -positive breast carcinomas evidenced that patients displaying an ATM-p+/HER2+ phenotype presented the shortest DFS (P=0.001).Pvalues were calculated using the log-rank test. Full size table Figure 6: Kaplan–Meier estimates of disease-free survival for ATM-p/HER2 status. Kaplan–Meier curves in a series of 167 HER2-negative and -positive breast carcinomas evidenced that patients displaying an ATM-p+/HER2+ phenotype presented the shortest DFS ( P =0.001). P values were calculated using the log-rank test. Full size image Several proteins, including Myc and PML, were originally identified as oncogenes or as tumour suppressors, according to their role in cancer and more precisely, to their gain of function or loss of function in the neoplastic state. However, a dualism in the function of these factors was later reported depending on the specific context, suggesting that this strict classification should be revised [38] , [39] , [40] . Here, we provide the first experimental demonstration for the tumorigenic potential of ATM activity, supporting the conclusion that ATM kinase, classically considered to be a tumour suppressor gene, may exert dual functions in cancer depending on the specific context. We show that ATM inhibition correlates very well with attenuation of HER2-dependent tumorigenicity and downstream signalling in vitro and in vivo . Furthermore, ATM phosphorylation identifies a subset of patients diagnosed with invasive HER2+ breast cancer characterized by significantly reduced DFS, so supporting ATM activity’s having a tumorigenic role in this context. Overall, these data suggest that ATM modulation may be successfully exploited to enhance the efficacy of therapeutic strategies. Our finding was unexpected since ATM heterozygosity has been proposed as a moderate predisposing factor for breast cancer risk, in line with the idea that ATM acts as a tumour suppressor gene. Interestingly, we observed that ATM-p-negative tumours are also preferentially HER2 negative ( Table 1 ). ATM does not significantly impact on the tumorigenicity of those hitherto analysed breast cancer cell lines, which either do not overexpress HER2 ( Fig. 1 ; Supplementary Fig. 2 ) or were transformed by other oncogenes such as RasV12 ( Fig. 1 ); both findings support the idea that ATM exerts its duality depending on the specific tumour context. Future experiments will further clarify whether ATM activity also sustains the oncogenic signals triggered by other HER family members or by other RTKs. We identified a molecular mechanism for ATM ability to modulate HER2 ( Fig. 5 ). ATM promotes the interaction between HER2 and HSP90 ( Fig. 4 ; Supplementary Fig. 7 ), a chaperone protein that is the main modulator of HER2 protein stability identified hitherto (reviewed in ref. 32 ), therefore preventing HER2 ubiquitination and degradation ( Fig. 4 ). Interestingly, proteomic studies previously identified HSP90 as a novel substrate of ATM in response to DNA damage [41] ; this raises the question of whether ATM may directly modulate HSP90 activity and also impinge on the stability of other HSP90 target proteins. We cannot rule out that additional mechanisms may also allow ATM to modulate HER2 levels and HER2 tumorigenicity. Trastuzumab, a humanized mAb directed against the extracellular domain of HER2, has radically improved the fate of HER2+ breast cancer patients; associated with chemotherapy, it is currently the mainstay of treatment of HER2-positive tumours both in the (neo)-adjuvant and metastatic settings. To better understand the relationship between ATM activation and HER2 positivity, we selected a series of patients treated for breast cancer in the pre-trastuzumab era. Therefore, none of the HER2+ breast cancer patients included in the study were treated with anti-HER2-targeted therapy. According to our hypothesis, ATM-p may indeed identify a subset of aggressive breast cancers characterized by high levels of HER2 expression/function ( Fig. 6 ) [22] . Despite the benefits shown by the introduction of Trastuzumab, a percentage of HER2-positive patients are intrinsically resistant or may develop resistance to this treatment. Multiple mechanisms have been proposed as contributing to Trastuzumab resistance [22] . We observed that ATM downregulation may significantly dampen Trastuzumab sensitivity ( Fig. 5 ), while conversely it may sensitize ER/HER2-positive cells to tamoxifen treatment ( Fig. 5 ). Future studies will clarify whether ATM-p provides a novel prognostic/predictive parameter and so plays a role in modulating HER2-positive tumour response to different therapeutic approaches. In summary, we propose that HER2-positive tumours have a selective advantage in retaining ATM expression/function. Our findings point towards a dual function of ATM in tumorigenesis and suggest that the status of ATM expression/activity may have real potential in improving both prognosis and therapy. Antibodies and reagents The following antibodies and reagents were used: anti-phospho-Ser1981-ATM (Cell Signaling, 1/500), anti-ATM (2C1; Santa Cruz Biotechnology 1/1,000), anti-tubulin (Sigma 1/3,000), Mouse anti-c-ErbB-2 protein monoclonal antibodies, clone TA-1 (anti-c- neu , Ab-5, Oncogene Science, for immunoprecipitations, 2 μg for 1 mg total extracts) and clone 3B5 (Ab-3, Oncogene Science, for western immunoblots, 1/1,000), anti-Ub ( P4D1 , Santa Cruz Biotechnology, 1/500), anti-Hsp90 (F8, Santa Cruz Biotechnology, 1/10,000), Anti-pS473-AKT (Cell Signaling, 1/1,000), anti-AKT (Cell Signaling, 1/1,000), anti-ATM (Ab-3, for immunoprecipitation, Oncogene Science, 2 μg for 1 mg total extracts), anti-Pan-Ras (Ab-3, Calbiochem, 1/1,000), anti-Neu (C-18, Santa Cruz Biotechnology, 1/1,000). Adriamycin (Sigma), CHX (Sigma) and KU-55933 (Calbiochem) are all commercially available. Trastuzumab (Herceptin) and Lapatinib were kindly provided by Regina Elena National Cancer Institute (Rome, Italy), 17AAG was kindly provided by D. Trisciuoglio and D. Del Bufalo. DNA constructs The pcDNA3–HER2 construct was kindly provided by P. Nisticò and the shATM construct by Y. Lerenthal and Y. Shiloh [42] . Control shRNA, siR5, has been described [43] . ATM was silenced by retroviral- or lentivirus-mediated expression of shRNA using pRETRO-Super vector [42] or pSIN18.cPPT.RNAi. p.EGFP.WPRE lentiviral vector [44] . Retroviral vectors pBabe, pBabe-H-RasV12 and pBabe-NeuT, constitutively active HER2 mutant (NeuV664E), for stable gene expression were kindly provided by M.J. Reginato [30] . HER2 was silenced by lentivirus-mediated expression of shRNA using pCCLsin.PPT.hPGK.GFP.Wpre vector [45] was kindly provided by S. Giordano. Cell cultures and infections All cell lines were grown at 37 °C in a CO 2 incubator (5%). Breast cancer cell lines MCF7, SKBR3, BT474 and T47D were kindly provided by Dr O. Segatto, ovarian cancer cell lines SKOV3 and non-transformed epithelial cell line MCF10A by F. Moretti and MCF7-pCDNA and MCF7-HER2 cell lines by P. Nisticò [46] . MCF10A cells were cultured using the MEGM Bullet Kit (CC-3150, Euroclone). HEK293T cell line was cultured as previously described. All other cell lines were cultured in RPMI-1640 containing 2 mM L -glutamine and supplemented with 10% HyClone* fetal bovine serum (Invitrogen). Retroviruses and lentiviruses were produced in HEK293T cells by cotransfecting pRETRO-Super and pSIN18.cPPT.RNAi. p.EGFP.WPRE lentiviral vector together with respective plasmids encoding for gag-pol and VSV-G proteins. Viral supernatants, collected 48 h post transfection, filtered through a 0.45-μm pore size filter, were added to the cells in the presence of 2 μg ml −1 polybrene. Forty-eight hours post infection with the retrovirus construct, cells were selected by 1 μg ml −1 of puromycin. Immunoprecipitations and immunoblotting Total cell extracts were prepared in lysis buffer (50 mM Tris-HCl, pH 7.5, 250 mM NaCl, 1% NP40, 5 mM EDTA, 5 mM EGTA, 1 mM phenylmethylsulfonyl fluoride, 25 mM NaF, 1 mM orthovanadate, 40 mM beta-glycerophosphate,10 mg ml −1 TPCK, 5 mg ml −1 TLCK, 1 mg ml −1 leupeptin, 10 mg ml −1 soybean trypsin inhibitor and 1 mg ml −1 aprotinin). For immunoblotting, 50 μg protein extract were separated by SDS–polyacrylamide gel electrophoresis, blotted onto nitrocellulose membrane and detected with specific antibodies [47] . HER2 receptor was immunoprecipitated from 2 mg of protein using anti-ErbB2 (c-Neu; Ab-5; Oncogene Science) and protein A-sepharose beads (Amersham). In the case of coimmunopreciptation experiments, cells were lysed in TMNS buffer (50 mM Tris-HCl, 150 mM NaCl, 20 mM NaMoO 4 , 0.09% NP40, 1 mM phenylmethylsulfonyl fluoride, 25 mM NaF, 1 mM orthovanadate, 40 mM beta-glycerophosphate, 10 mg ml −1 TPCK, 5 mg ml −1 TLCK, 1 mg ml −1 leupeptin, 10 mg ml −1 soybean trypsin inhibitor and 1 mg ml −1 aprotinin ), while for the ubiquitination assay cells were lysed with RIPA buffer (50 mM Tris pH 8, 150 mM NaCl, 1% NP40, 0.1% SDS, 0.5% NaDeoxycolate, plus 20 mM NEM (Sigma E1271), 1 mM phenylmethylsulfonyl fluoride, 25 mM NaF, 1 mM orthovanadate, 40 mM beta-glycerophosphate,10 mg ml −1 TPCK, 5 mg ml −1 TLCK, 1 mg ml −1 leupeptin, 10 mg ml −1 soybean trypsin inhibitor and 1 mg ml −1 aprotinin). Analysis of HER2 receptor levels To analyse the expression of HER2 receptor, cells were incubated for 30 min at room temperature with mouse anti-HER2 Ab-5 antibody. Cells were then reacted with phycoerythrin-conjugated goat anti-mouse IgG (H-L) (Pharmingen) for 30 min at room temperature. Cells were analysed by flow cytometry. Mean fluorescence intensity of cells stained with anti-HER2 was used to compare the level of HER2 expression, calculated with % of difference in mean fluorescence intensity in different conditions with respect to control isotype. Flow cytometry of phospho-Ser1981-ATM Cells (5 × 10 5 ) were fixed in 4% formaldehyde, incubated for 15 min at 4 °C, permeabilized by resuspending in 1 ml ice-cold MeOH and incubated at −20 °C overnight (O/N). Cells were resuspended in PBS-Tween 0.5% containing 5% normal goat serum containing anti-mouse phospho-Ser1981-ATM (Cell Signaling) primary antibody, incubated for 1 h at room temperature and incubated with anti-mouse AlexaFluor488-conjugated secondary antibodies. Mean fluorescence intensity of cells stained with anti-pS1981-ATM was used to compare the level of pS1981-ATM expression (ATM-p) calculated with % of difference in mean fluorescence intensity in different conditions compared with control isotype (FACScanto, Becton Dickinson) as described [47] . Briefly, cells were fixed in 4% formaldehyde and incubated 15 min at 4 °C. They were then permeabilized by resuspending with vigorous vortexing in 1 ml ice-cold MeOH and incubated at −20 °C O/N. Cells were washed and resuspended in PBS-Tween 0.5% containing 5% normal goat serum containing anti-mouse-phospho-Ser1981-ATM and incubated for 1 h at room temperature. After washing and repeating the process with anti-mouse-AlexaFluor488-conjugated secondary antibodies, flow cytometry was evaluated in a FACScanto (Beckton Dickinson). Cell proliferation assay MCF10A-pBabe, MCF10A-pBabeshATM, MCF10A-NeuT, MCF10A-NeuT-shATM, MCF10A-RasV12, MCF10A-RasV12shATM cells were maintained for 72 h in Dulbecco’s modified Eagle’s medium/F-12 supplemented with 1% FBS. All cell lines were seeded in triplicate in six-well plates at a density of 8 × 10 4 cells per well in the same medium. Survival and anchorage-independent growth For survival assays, MCF7-HER2 cells were seeded in a serum-free medium; Trastuzumab was applied 24 h later. Viability was assessed 72 h after treatment, with the Cell Titer GloLuminescent Assay (Promega). Anchorage-independent growth assays were performed as described [48] . Data on biological assays are representative of three independent experiments performed in triplicate. In vivo tumorigenesis assays All procedures involving animals and their care were conducted in conformity with the institutional guidelines. This study has been reviewed and approved by the ethics committee of the Regina Elena National Cancer Institute. Xenografts from MCF7-HER2 cells were obtained on 40-day-old SCID female mice (Harlan Laboratories, Udine, Italy). At day 0, SCID mice were fully anesthetized and 17-h estradiol pellets were subcutaneously injected. The day after, 5 × 10 6 exponentially growing MCF7-HER2 cells were mixed 1:1 with Matrigel (BD Biosciences, San Jose, CA, USA) and injected subcutaneously as previously described [48] . Tumour development was followed twice a week by caliper measurements along two orthogonal axes: length ( L ) and width ( W ). The volume ( V ) of tumours was estimated by the formula V = L × ( W 2 )/2 (ref. 31 ). Three independent tumorigenesis assays were performed (total of 22 mice were used: 11 mice bearing MCF7-HER2 siR5 xenografts and 11 mice bearing MCF7-HER2-shATM xenografts). A transgenic mouse carrying the mutated rat HER2/ neu oncogene driven by the MMTV promoter [31] was mated with FVB females (Charles River, Calco, Italy). The progeny was screened for the transgene by PCR. Transgene-carrying females were backcrossed with FVB males for 12 generations and HER2/ neu + FVB mice (FVB–NeuT) were used in these experiments. Females of transgenic lines show a MMTV-driven overexpression of the transgene in the mammary gland and a definite tumour growth involving the mammary gland epithelium [31] . Starting at the age of 13 weeks after birth, their mammary glands were inspected once a week and upon development of the first tumour, we injected intraperitoneally KU-55933 at the 10 mg kg −1 concentration (6 animals) or dimethylsulphoxide (6 animals) as control every 2 days for 2 weeks. Tumour growth was monitored by measuring using calipers in the two perpendicular diameters, and tumour volume calculated as described above and according to Boggio et al. [31] . Patients The 167 cases included in the study consisted of a series of 87 (52.1%) HER2-positive primary breast carcinomas and a control series of 80 (47.9%) HER2-negative primary breast carcinomas collected from the surgical pathology files of the Regina Elena National Cancer Institute. Patients have been fully described in Supplementary Methods and Tables . Tumours were graded according to Bloom and Richardson and staged according to the Unione Internationale Contre le Cancer tumor-node-metastasis system criteria and histologically classified according to the World Health Organization [49] . Follow-up data were obtained from hospital charts and by corresponding with the referring physicians. Patients had a median follow-up of 53 months (range: 3–124). This study was reviewed and approved by the Ethics Committee of the Regina Elena National Cancer Institute. Informed written consent was obtained from all the subjects. Immunohistochemistry Formalin-fixed paraffin-embedded tissues from multiple breast cancer from seven FBV-NeuT mice and from 167 human breast carcinomas were cut on SuperFrost Plus slides (Menzel-Glaser, Braunschweig, Germany). Two-micron-thick sections were stained with a streptavidin-enhanced immunoperoxidase technique (Supersensitive Multilink, Novocastra, Leica, Italy) in an automated autostainer (Bond Max, Leica) using the ATM-p mAb (clone 7C10D8, Rockland, tebu-bio, Italy), and a pH-6 citrate buffer antigen retrieval protocol. ATM-p was considered as positive when at least 10% of the neoplastic cells showed a nuclear/cytoplasmic immunoreactivity. In the 167 human breast cancer samples, ER and PgR status as well as HER2 and Ki67 were assessed by IHC as described above. Scoring criteria are reported in Supplementary Methods . Evaluation of the immunohistochemical results was performed independently by two investigators (M.M. and A.D.B.). Statistical analysis All experiments were performed at least three times for statistical significance. Numerical data were expressed as mean+s.d. Statistical analysis was performed using the Student’s t -test, P <0.05 being considered significant. Quantification of tumour growth in mice was analysed by a two-tailed Student’s t -test. A P <0.05 was considered as significant. Statistical analysis was carried out using the Analyse-it software for Microsoft Excel (Analyse-it Software Ltd, Leeds, UK, version 1.62). For immunohistochemistry experiments on a primary tumour sample, the associations were tested by the Pearson χ 2 -test or Fisher exact test when appropriate. P values <0.05 denote statistically significant associations. DFS curves were estimated by the Kaplan–Meier method. Additional information is detailed in Supplementary Methods . How to cite this article: Stagni, V. et al. ATM kinase sustains HER2 tumorigenicity in breast cancer. Nat. Commun. 6:6886 doi: 10.1038/ncomms7886 (2015).